Continuous adsorption in highly ordered porous matrices made by nanolithography The exposed surface area of porous materials is usually determined by measuring the mass of adsorbed gas as a function of vapour pressure. Here we report a comprehensive study of adsorption in systems with closed bottom, not interconnected pores exhibiting different degrees of disorder, produced with methods encompassing nanolithography and dry and wet etching. Detailed adsorption studies of these matrices show hysteresis loops, as found always in pores having sizes of tens to hundreds of nanometres. The observed variations in the loop shape are associated with changes in the pore morphology. In regular pores formed by vertical and smooth walls, continuous adsorption is found for the first time in agreement with thermodynamic considerations valid for ideal pores. This suggests that irregularities in the walls and pore openings are the key factors behind the hysteresis phenomenon. Interestingly, pores having rough walls but a pyramidal shape also do not show any hysteresis. Porous solids represent a broad class of natural and synthetic materials that find many applications in a variety of different fields, ranging from catalysis to oil extraction and from mixture separation to pollution control [1] , [2] . They all share complicated pore connectivity and a broad distribution of pore sizes, whose mean value ranges from nanometre-to-micron size, depending on the material. Advances in nanotechnology have made possible the realization of self-assembled porous materials, which present uniform arrays of straight, non-connected pores, following fairly simple methodologies. Examples of such materials include silica SBA-15 (ref. 3 ) and MCM-41 (ref. 4 ), porous alumina [5] , [6] and silicon [7] . Because of their regularity, these matrices have been exploited as templates for the realization of new functional materials [8] , [9] , [10] . One of the key parameters of all porous materials is the total surface area exposed to a gas. The only method to determine it relies on the measurement of adsorption isotherms [1] , [2] . These curves represent the mass of the gas, typically N 2 or Ar at liquid nitrogen temperature, adsorbed onto a substrate as a function of the equilibrium vapour pressure of the surrounding vapour. In the case of porous materials having pores ranging from 10 to 100 nm in size, they always exhibit two main features: (i) a sharp increase in the amount of adsorbed gas well below the liquid–vapour coexistence pressure P 0 of the bulk adsorbate, which is explained in terms of capillary condensation in the small pores [11] , [12] . Below a certain pressure, a film covers uniformly the inner walls of the cavity, whereas above it the cavity fills up completely with liquid, even though that phase is not thermodynamically stable in bulk; (ii) a hysteresis loop between the adsorption (gas is added to the sample cell) and the desorption (gas is removed from the sample cell) branches. Condensation occurs at a pressure P ads larger than the pressure of evaporation P des . As the pore size increases, both these quantities move closer to P 0 . Despite its commonplace occurrence, the origin of the hysteresis phenomenon is still a matter of debate [12] , [13] . According to macroscopic thermodynamic arguments [14] , the hysteresis is usually explained in terms of the different shape of the vapour/adsorbate interface during adsorption and desorption in a cylindrical pore with open ends [1] , [2] . This implies that in the case of a cylindrical pore with only one open end, no hysteresis is expected because the meniscus nucleates at the bottom corners and is the same, both in adsorption and in desorption. Mean density functional theory [15] , molecular dynamics simulations of adsorption and desorption by diffusive mass transfer into model pores [16] and grand canonical Monte Carlo simulations [17] confirm this classical picture of adsorption in a single pore. In contrast to theoretical predictions, experiments with mesoporous matrices characterized by a trivial porous network topology consisting of straight and not interconnected pores show that adsorption is always characterized by pronounced hysteresis loops independent of whether the pores are open at one or at both ends [7] , [12] , [18] , [19] , [20] , [21] . In other words, in these materials the pores appear not to be independent during an adsorption isotherm. Over the years, various mechanisms have been suggested to explain pore coupling, including the presence of a thin planar liquid film around the pore openings connecting adjacent pores during desorption [7] , [22] , elastic deformations of the porous matrix in adsorption–desorption [23] , quenched disorder imposed by some variation of the pore diameter along the pore axis [24] , [25] and of the fluid/wall interaction [26] . More recently, detailed simulations [27] in a uniform closed-bottom pore show hysteresis and the causes are attributed to a variation in the shape of the meniscus and the change in the packing of the adsorbate during adsorption and desorption, which are not accounted for in classical theories. Here we show that in contrast to previous experimental evidences and to the conclusions of theories trying to rationalize the systematic occurrence of hysteresis, in very regular closed-bottom pores formed by vertical and smooth walls no hysteresis in adsorption isotherms is observed, in agreement with the thermodynamic considerations valid for ideal pores. Nanofabrication of porous matrices To experimentally elucidate this problem, we have fabricated by advanced nanofabrication a series of arrays of closed-bottom, non-interconnected pores, with a characteristic size of ∼ 100 nm and with different levels of morphological disorder. Adsorption isotherms measured in pores presenting bottlenecks and variations in size along the pores show the typical hysteresis loops. However, in regular pores with (i) uniform cross-section, (ii) vertical sidewalls and (iii) nearly atomic-scale surface roughness, adsorption is found to be reversible as expected by thermodynamic arguments, indicating that morphological disorder is the ultimate cause of the observed hysteresis. Although modern dry-etching technologies have enabled the realization of high aspect-ratio nanostructures with almost vertical and smooth sidewalls into various materials, the stringent criteria (i–iii) can be fulfilled only approximately. Therefore, a more elaborated process was designed for the fabrication of porous samples satisfying all the above specifications. The key idea behind the overall fabrication process, depicted in Fig. 1 , consists of using nanoimprint lithography (NIL) [28] , [29] and dry-etching techniques to form an array of holes into (110)-oriented crystalline silicon, followed by anisotropic wet etching in an alkaline solution that expands the holes previously obtained until these become delimited by {111} planes. It is well known that {111} planes, with one dangling and three covalent bonds per atom, are extremely slow-etching planes in alkaline solutions, up to two orders of magnitude slower than other low-index crystal planes with smaller (larger) number of covalent (dangling) bonds per atom. The large etch-rate anisotropy makes {111} planes behave almost as etch stops. With the choice of the (110)-oriented crystalline silicon substrate, two of the {111} planes, namely the and the , are orthogonal to the substrate surface. Therefore, the holes created in the first step of dry etching evolved ( Fig. 1A , steps j and k) during the anisotropic wet etching towards a parallelepiped delimited on the sides by couples of and crystallographic planes (which correspond to a parallelepiped of rhombic cross-section). The pores are delimited at the bottom and at the top by and planes. However, although the bottom of the pores ends at the intersection line between and (111) planes, the two planes delimiting the pores at the top do not intersect, being truncated by the presence of the opening in the initial lithographically defined tungsten/nickel mask. The wet-etching step produces nearly atomically flat {111} planes, with the effect of ‘healing’ the imperfections and surface roughness of the nanostructures obtained after the dry-etching step. The pattern of the porous matrices was defined by NIL. This technique essentially consists of moulding the features of a stamp into a thin polymer film when this, by proper setting of the temperature, is in the melting state and is free to flow. After indentation of the stamp features, the complementary features in the polymer can be frozen into their shape by cooling the temperature down below the polymer glass transition temperature. The choice of NIL technique was made because it allows an excellent reproduction of nanometric-scale features [28] and the fast and parallel patterning of macroscopic areas (≥1 cm 2 ), as needed to fall within the sensitivity range of the chosen gravimetric detection scheme based on the use of a torsional microbalance. 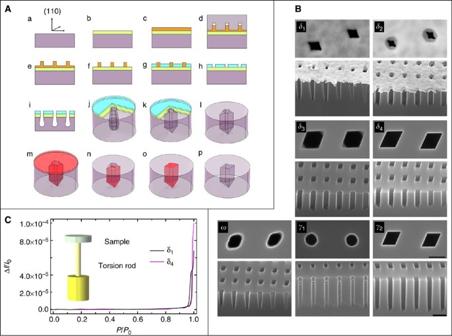Figure 1: Nanofabrication of porous matrices and gravimetric measurement of isotherms. (A) Fabrication of the porous matrices. (B) SEM images of the top and cross-sectional views of various pores produced in this study. (C) Complete adsorption isotherms of Ar atT=85 K for two porous samples, and the scheme of the torsional microbalance used for the measurements. (A) Double-side-polished (110)-oriented silicon (a) is sputtered (b) with 40 nm of tungsten. (c) A resist film is spin coated and patterned with a pillars’ array by NIL (d,e), using different stamps for the seriesδandγ(Supplementary Figs S1 and S2). (f) Residual resist layer is etched by oxygen plasma, exposing the tungsten underneath and reducing controllably the vertical and lateral size of nanopillars. (g) Forty-nanometre hard nickel mask is electroplated on tungsten, following established process strategies31. (h) The resist is stripped in acetone. (i) The pattern is transferred from nickel into tungsten and silicon by reactive ion etching, either with continuous (δ-series) or time-multiplexed processes (γ-series; see Methods). (k) Holes of non-uniform cross-section, rough and sloped sidewalls (j) are ‘healed’ by wet anisotropic etching in aqueous tetramethylammonium hydroxide (TMAH), resulting in holes of rhombic cross-section delimited byandplanes, and capped at both ends byandplanes, and by the opening in the tungsten/nickel mask. (l) The hard nickel mask is lifted by etching the tungsten underneath in H2O2. The holes’ bottleneck (formed by re-entrant planesand) is removed by steps (m–p). (m) Polymethyl methacrylate (PMMA) is spin coated to protect the holes and is back-etched by oxygen plasma. (o) The bottlenecks are dry etched without affecting the inner pores’ surface protected by PMMA, which is subsequently dissolved in acetone (p). (B)δ- andγ-series were generated by stopping fabrication at different steps.δ1,δ2,δ3andδ4result from stepsj,k,l,p, respectively.γ1andγ2were obtained by Bosh process at stepi.γ1exhibits restrictions (‘scallops’) along the depth of the pores, whereasγ2was processed up to stepp. The tungsten/nickel mask was removed after stepjfor samplesγ1andω. Scale bars, 200 nm for top-view and 500 nm for cross-view images. Figure 1: Nanofabrication of porous matrices and gravimetric measurement of isotherms. ( A ) Fabrication of the porous matrices. ( B ) SEM images of the top and cross-sectional views of various pores produced in this study. ( C ) Complete adsorption isotherms of Ar at T =85 K for two porous samples, and the scheme of the torsional microbalance used for the measurements. ( A ) Double-side-polished (110)-oriented silicon ( a ) is sputtered ( b ) with 40 nm of tungsten. ( c ) A resist film is spin coated and patterned with a pillars’ array by NIL ( d , e ), using different stamps for the series δ and γ ( Supplementary Figs S1 and S2 ). ( f ) Residual resist layer is etched by oxygen plasma, exposing the tungsten underneath and reducing controllably the vertical and lateral size of nanopillars. ( g ) Forty-nanometre hard nickel mask is electroplated on tungsten, following established process strategies [31] . ( h ) The resist is stripped in acetone. ( i ) The pattern is transferred from nickel into tungsten and silicon by reactive ion etching, either with continuous ( δ -series) or time-multiplexed processes ( γ -series; see Methods). ( k ) Holes of non-uniform cross-section, rough and sloped sidewalls ( j ) are ‘healed’ by wet anisotropic etching in aqueous tetramethylammonium hydroxide (TMAH), resulting in holes of rhombic cross-section delimited by and planes, and capped at both ends by and planes, and by the opening in the tungsten/nickel mask. ( l ) The hard nickel mask is lifted by etching the tungsten underneath in H 2 O 2 . The holes’ bottleneck (formed by re-entrant planes and ) is removed by steps ( m – p ). ( m ) Polymethyl methacrylate (PMMA) is spin coated to protect the holes and is back-etched by oxygen plasma. ( o ) The bottlenecks are dry etched without affecting the inner pores’ surface protected by PMMA, which is subsequently dissolved in acetone ( p ). ( B ) δ - and γ -series were generated by stopping fabrication at different steps. δ 1 , δ 2 , δ 3 and δ 4 result from steps j , k , l , p , respectively. γ 1 and γ 2 were obtained by Bosh process at step i . γ 1 exhibits restrictions (‘scallops’) along the depth of the pores, whereas γ 2 was processed up to step p . The tungsten/nickel mask was removed after step j for samples γ 1 and ω . Scale bars, 200 nm for top-view and 500 nm for cross-view images. Full size image Not all samples were obtained following the whole procedure just described. To identify how the changes in the pore morphology reflect into the shape of adsorption isotherms, from batches of substrates processed in the same conditions, we picked out samples at different stages of the process flow. Samples of the δ -series and sample ω , whose top and cross-view electron micrographs are presented in Fig. 1B , were obtained using a nanoimprinting stamp (used in the process in Fig. 1A , step d; scanning electron microscopy (SEM) micrograph is shown in Supplementary Fig. S1 ) with arrays of holes of rhombic cross-section and a continuous dry-etching process of silicon (process Fig. 1A , step i). The sample ω corresponds to step i after the removal of the metal mask. The fabrication of samples δ 1 , δ 2 , δ 3 and δ 4 were stopped at stages j (leaving the metal mask), k, l and p, respectively. The samples of the γ -series were obtained using a nanoimprinting master with arrays of cylindrical holes ( Supplementary Fig. S2 ) and a time-multiplexed, deep, reactive ion-etching process (at Fig. 1A , step i), alternating a nearly isotropic etching step based on sulphur hexafluoride (SF 6 ) to passivation steps based on octafluorocyclobutane (C 4 F 8 ) [30] . This process (also referred to as Bosch process) is known to produce ‘scallops’, that is, nearly periodic undulations on the sidewalls with characteristic periodicity of 50–500 nm. It was introduced on purpose to test the effect of restrictions in the pores and to produce pores of higher aspect ratio. The samples that were etched only by a dry process present a surface roughness whose upper limit is estimated to be 3 nm (root mean square (r.m.s.)). For all other samples whose surface was smoothed by the wet-etching step, the r.m.s. roughness is guessed to be well below 1 nm. In both cases, the surface is chemically uniform and no variations in the fluid/wall interaction are expected. Further details on the fabrication and characterization of the samples are presented in Methods and Supplementary Table S1 . Adsorption isotherms We have measured adsorption isotherms with a torsional microbalance [32] . The porous samples, having a characteristic size of ∼ 1 cm and a thickness of a few hundred microns, are attached to the extremity of a tungsten rod driven to its torsional frequency by means of piezoelectric crystals (see inset of Fig. 1 ). As the samples are exposed to a vapour of argon at T =85 K, the resonance frequency decreases because of an increase in the total moment of inertia. From the vapour-corrected frequency shifts, it is then possible to derive the relative change of the oscillator moment of inertia, Δ I / I 0 , which is proportional to the mass of the adsorbed film [32] . The graph of Fig. 1 shows two typical adsorption isotherms taken with the nanopatterned samples. They present negligible adsorption apart from a very steep and big step occurring close to saturation due to the capillary filling of the pores. The higher final value of the isotherm δ 4 reflects the larger pore volume of this sample. More important, isotherm δ 1 shows hysteresis, whereas δ 4 is reversible. 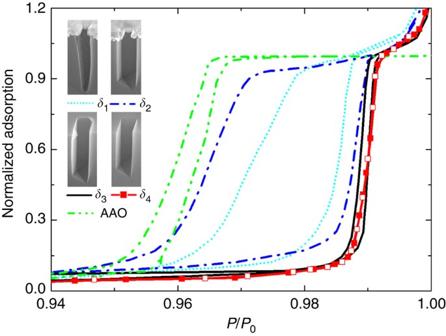Figure 2: Adsorption isotherms near condensation pressure on the nanopatterned silicon samples. The adsorption data are normalized to the values of the plateaus observed after capillary condensation. The SEM micrographs show representative cross-sections of the various pores. The curves are compared with previously published adsorption isotherms in mesoporous alumina (AAO)21. Figure 2 shows a sequence of adsorption isotherms taken with a series of δ -samples. To facilitate their comparison, the data are displayed in a much enlarged scale close to saturation and the adsorption data have been normalized to the values of the plateaus observed after capillary condensation. The isotherm of δ 1 is characterized by a pronounced hysteresis loop between the adsorption and the desorption branches, which reflects the pore morphology. This sample features pores of tapered shape with an open mouth of ∼ 180 nm, a closed bottom of ∼ 90 nm and rough inner surface. At the top, the pores present bottlenecks due to the metallic mask. Hysteresis is then likely to be due to the presence of bottlenecks and irregular, rough walls. Its shape resembles that of type H1 in the IUPAC classification [33] (for example, a hysteresis loop with parallel adsorption and desorption branches), which is generally associated with capillary condensation and evaporation in ordered mesoporous materials with cylindrical pores. As a reference, the same graph shows the isotherm taken in mesoporous alumina with closed-bottom pores having a circular cross-section with a diameter of ∼ 60 nm but no bottlenecks, published some time ago [21] , whose loop resembles that observed with δ 1 . The fact that the loop of δ 1 is shifted to higher pressures is simply because of the larger pores of δ 1 . Instead, the significant widening of the loop is likely to be due to the presence of bottlenecks and rough walls in the δ 1 pores [34] . Figure 2: Adsorption isotherms near condensation pressure on the nanopatterned silicon samples. The adsorption data are normalized to the values of the plateaus observed after capillary condensation. The SEM micrographs show representative cross-sections of the various pores. The curves are compared with previously published adsorption isotherms in mesoporous alumina (AAO) [21] . Full size image Interestingly, a wider hysteresis loop opens up in the isotherm of sample δ 2 , featuring pores of nearly atomically flat inner walls and uniform cross-section. The pores are closed at the bottom by two oblique {111} planes and at the top end in a neck smaller than that of δ 1 . The slight shift of the condensation branch to higher P/P 0 reflects the enlargement to ∼ 250 nm of the pore cavities [35] in sample δ 2 , which occurred during the etching process k as compared with the average size of δ 1 . Instead, the shift of the evaporation branch to lower P/P 0 is likely to be caused by the smaller neck size. In fact, the smallest distance between the opposite edges of the neck opening deduced from SEM images of the top sample surfaces are 68±8 nm for sample δ 2 instead of 84±12 nm for sample δ 1 (see Supplementary Table S1 ). Both values are much larger than the critical size D c below which evaporation from the pore cavity occurs via cavitation. In fact, D c is ∼ 5 nm for N 2 in porous silica [35] and D c ∼ 4 nm for Ar in porous carbon [34] . Accordingly, desorption in samples δ 1 and δ 2 takes place via ‘pore blocking’, that is, there is a gradual decrease of the adsorbed liquid volume, which results when the meniscus recedes from the end of the necks and moves towards the interior of the pore [33] . The presence of rough walls may also affect the observed hysteresis loops. However, a quantitative analysis of this contribution is still lacking. In sample δ 3 , the top metal mask was stripped away and the restriction of the pore opening was much less pronounced, represented by two re-entrant {111} planes at the two opposite corners on the long axis of the rhombic cross-section. The graph of Fig. 2 shows that the hysteresis loop of the corresponding isotherm is found to shrink and shift to higher P/P 0 . Again, the shift can be explained as an enlargement of the pores by wet etching in step k; the pore cavity is ∼ 250 nm. Furthermore, the hysteresis is still likely to be caused by the restriction observed near the pore openings formed by the planes and (111). However, the loop is now narrower because the difference between the size of the pore cavity and that of the neck in δ 3 is significantly smaller than in the previous two samples. Finally, the regular pores of sample δ 4 present vertical, nearly atomically flat walls and the complete absence of any neck at the opening. The adsorption in this almost-ideal pore array yields a fully reversible curve. More accurately, the data set an upper limit to the hysteresis width, which must be smaller than ∼ 2 × 10 −4 in relative pressure, which corresponds to 0.1 Torr in absolute pressure. Our results confirm the thermodynamic argument of the absence of hysteresis in regular closed-bottom pores, although it is at variance with recent simulations [27] that find hysteresis in a cylindrical closed-bottom pore having a diameter of 7 nm and a length of 20 nm. We believe that this disagreement is simply due to the much larger pores of sample δ 4 used in the experiment (distance between parallel planes of the pores is ∼ 200 nm and length 400 nm). For such wide pores, the effects due to (i) the structural change of the adsorbate and (ii) the variation of the shape of the meniscus during adsorption should yield a negligible contribution. We have analysed the capillary jump of the δ 4 isotherm in terms of the classical Kelvin equation, which relates the quantity ln(P/P 0 ), corresponding to a liquid filling a cylindrical pore, to the curvature C of the meniscus [7] , [13] : where γ =13.1 erg cm −2 is the liquid argon surface tension and n liq =2.1 × 10 22 atoms per cc is the liquid argon number density, both evaluated at the temperature T =85 K, K B =1.38 × 10 −16 erg K −1 being the Boltzmann constant. For an ideal cylindrical pore closed at one end, the meniscus is expected to have the same hemispherical shape during condensation and evaporation [14] so that C =4/ D , where D is the pore diameter. As the capillary jump occurs in the interval P < / P 0 =0.986≤ P / P 0 ≤0.992= P > / P 0 with the midpoint at P mid-point / P 0 =0.9898, this analysis yields a mean diameter D =206 nm and a dispersion σ =9%D, assuming that D >,< =D ±3 σ , which is in substantial agreement with the distance ∼ 200 nm between the parallel walls derived from the real space images of the pores (see Supplementary Table S1 ). In fact, if we consider the crudity of the thermodynamic model employed and the complexity of the pore cross-section, this quantitative agreement is rather surprising. The sequence of δ isotherms suggests that the morphological disorder of the porous matrix is at the origin of the hysteresis phenomenon. To better clarify the role had by disorder, we have also prepared some other pores with different morphologies. 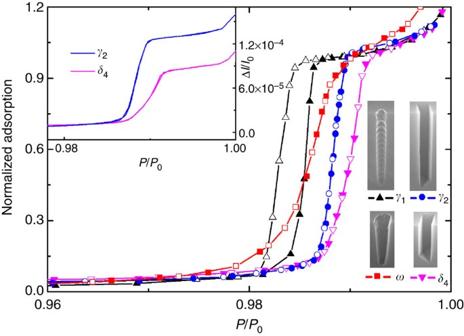Figure 3: Adsorption isotherms near condensation pressure on the nanopatterned silicon samples. The adsorption data are normalized to the values of the plateaus observed after capillary condensation. The SEM micrographs show representative cross-sections of the various pores. The inset compares the variation of the moments of inertia measured along the capillary jumps in samplesγ2andδ4. Figure 3 shows the cross-section of the pores of sample γ 1 . They were obtained by dry etching with a ‘Bosch process’ (known also as pulsed or switched process), alternating passivation and etching steps, leading to the formation of ‘scallops’, that is, (almost) periodic re-entrances along the etching direction. The pore-size first oscillations are between 128±8 and 156±9 nm, and the open mouth is 135±6 nm. The corresponding isotherm in Fig. 3 shows a narrow loop of type H1. We have found similar loops in modulated alumina pores having a different number N of large domains ( D =35 nm) alternated by narrow ones ( D =25 nm) [36] . Both the experimental and simulation data showed that capillary condensation and evaporation were driven by the smallest size of the nanopore (constriction). Figure 3: Adsorption isotherms near condensation pressure on the nanopatterned silicon samples. The adsorption data are normalized to the values of the plateaus observed after capillary condensation. The SEM micrographs show representative cross-sections of the various pores. The inset compares the variation of the moments of inertia measured along the capillary jumps in samples γ 2 and δ 4 . Full size image The sample γ 2 is instead the most regular sample we managed to make. It has smooth pores of rhombic cross-section defined by {111} planes produced in the same way as δ 4 . The parallel vertical sidewalls are separated by a mean distance of ∼ 185 nm, slightly smaller than the 195 nm of δ 4 , but the pores are significantly longer: 985±22 nm instead of 640±17 nm ( Supplementary Table S1 ). These differences are reflected in the shape of the capillary rises plotted in terms of the absolute adsorbed amount in the inset of Fig. 3 . First of all, both curves are fully reversible because the closed-bottom pores are highly uniform. Next, the jump of γ 2 occurs at slightly lower relative pressures because the pores are smaller in cross-section. Similarly, the capillary rise of γ 2 is much steeper, indicating a narrow distribution of pore sizes. In fact, its analysis in terms of the Kelvin equation [37] yields a mean diameter D =180 nm and a dispersion σ =6% D , which, again, agrees very well with the SEM analysis ( Supplementary Table S1 ) and is smaller than the best values obtained with porous alumina or silica [21] . Finally, the inset of Fig. 3 indicates that the amount of gas filling the pores of sample γ 2 is ∼ 1.5 larger than that of δ 4 because the pores are longer, and this factor coincides with the ratio of the pore heights as deduced from the SEM analysis. Interestingly, a rough inner surface of the pores does not necessarily imply adsorption hysteresis as shown by the sample ω , which features pores of non-uniform cross-section having walls with a roughness of ∼ 3 nm. The pores, having a height of ∼ 700 nm, are obtained only by dry etching (without wet etching), after the removal of the hard mask. The pores opening at the top has a mean value of 160±9 and 167±12 nm for the minimum distances between opposite edges and the cross-section is tapered down to a width of 91±10 nm. The isotherm is reversible, although the capillary jump is less steep than those of the samples γ 2 and δ 4 . The broader jump is related to the varying size of the cross-section. In fact, if this jump is analysed in terms of the Kelvin equation as discussed above, we find a mean diameter D =140 nm and a dispersion σ =15% D . As for the absence of hysteresis, we do not have a clear explanation and we urge the theorists to analyse adsorption in conical or pyramidal pores. In summary, we have fabricated a series of nanopatterned samples formed by arrays of closed-bottom pores where the morphological disorder is varied in a controlled way. Detailed adsorption studies carried out in these matrices show the typical hysteresis loops that are always found in pores having a characteristic size of the order of tens of nanometres. The observed variations in the loop shape have been associated to changes in the pore morphology. The novel result is the finding of fully reversible adsorption in very regular pores formed by vertical and smooth walls in agreement with thermodynamic considerations valid for an ideal pore. This suggests that the irregularities in the walls and in the pore openings present in natural and synthetic porous materials are the key factors behind the commonly observed hysteresis phenomenon, at least for pores having a size comparable to that in this study ( ∼ 200 nm). Interestingly, pores having rough walls but a pyramidal shape, that is, with a strictly monotonic dependence of the cross-sectional area from the closed bottom end to the top mouth, also do not show any hysteresis. Fabrication of the NIL stamps The fabrication of γ - and δ -series involved the use of NIL. The pattern of the stamps was derived, through different processes, from commercial periodic structures originated by interference lithography. In particular, in the fabrication of all samples of the γ -series, we used a single silicon stamp consisting of a square array of cylindrical holes, obtained by inverting the pattern of a square array of cylindrical pillars, by NIL and deep, reactive ion-etching. In the fabrication of the δ -series, we used as a stamp a sample with holes of rhombic cross-section. This was done according to the scheme of Fig. 1A (up to step p) and belonged to a preliminary series of samples whose adsorption isotherms are not reported in this work. The rationale of ‘feeding back’ a sample at the beginning of the fabrication process and using it as a stamp was to form already in the dry-etching step ( Fig. 1A , step j) holes of shape that better approximate the final rhombic cross-section resulting after wet etching. The shape of the bottleneck in the samples δ 1 and δ 2 , and the cross-section of the pores in samples δ 1 and ω reveal the initial rhombic shape of the holes in the stamp. Details of the fabrication of stamps and samples are reported below. Stamp for the γ-series . Silicon (100) wafers were diced into 3 × 3 cm 2 substrates and dehydrated on a hot plate at 150 °C for 10 min. A 260-nm-thick mr-I 7030E (Micro Resist Technology GmbH) resist film was applied by spin coating at 4,000 r.p.m. and annealed at 140 °C for 2 min on a hot plate. We obtained a stamp with holes by inverting by NIL the tone of a square array of cylindrical pillars (250 nm diameter, 300 nm height and 500 nm period) made by interference lithography and transferred to silicon. The stamp with pillars was functionalized with a monolayer of octadecyltrichlorosilane self-assembled from vapour phase as an anti-adhesion coating. Imprinting was performed at a 5.5-MPa pressure and 90 °C for 6 min. The residual layer of 20 nm was etched in oxygen plasma. The pattern was transferred by reactive ion etching in an inductively coupled plasma system with a process at 8 mTorr pressure, C 4 F 8 , SF 6 and Ar flows of 60, 30 and 10 s.c.c.m., respectively, and 400 and 20 W radio-frequency power applied to coil and platen, respectively, for 2 min. The remaining resist was removed by oxygen plasma. The resulting stamps, shown in Supplementary Fig. S1 and consisting of an array of holes (215 nm diameter, 250 nm of depth and period of 500 nm), were functionalized with an octadecyltrichlorosilane monolayer to improve its anti-adhesion properties. Stamp for the δ-series. The fabrication of the NIL stamp used for the nanopatterning of the δ- series was obtained by a process analogous to that used in the fabrication of samples γ 2 and δ 4 , that is, the entire process described in Fig. 1A , up to step p (as described in detail in the next section). This resulted in a stamp with the same rhombic cross-sectional shape of the measured samples. Fabrication of the samples of the γ - and δ -series Adsorption isotherms were measured on porous samples with accurately controlled morphology, fabricated by a combination of sputtering, NIL, electroplating, deep reactive etching and wet anisotropic etching on crystalline silicon as detailed below. Boron-doped Si (110) wafers, 4 inches in diameter, were diced into 3 × 3 cm 2 substrates, dehydrated on a hot plate at 150 °C for 10 min and coated with a 40-nm-thick tungsten layer by RF magnetron sputtering. A 90-nm-thick film of mr-I 8010E resist (Micro Resist Technology GmbH) was spin coated at 3,000 r.p.m. and annealed for 2 min on a hot plate at 140 °C. Two different NIL stamps were used for patterning the resist film by NIL for the γ - and δ -series (including the sample ω in the latter). The optimized NIL thermomechanical cycle was attaining 170 °C and 7.5 MPa as maximal values for temperature and pressure, respectively, conditions that were maintained for 8 min before cooling the temperature down to 50 °C and releasing the pressure. For the NIL process of the δ -series, the reciprocal orientation of stamp and sample, both on (110) silicon substrates, was controlled to have the main crystallographic planes aligned within 1°. The residual resist layer was removed by oxygen plasma, which allows to shrink laterally, in a controlled way, the resist nanopillars exploiting the isotropic component of the oxygen plasma process. The latter was performed at 4 mTorr pressure, RF power to platen and coil of 200 and 10 W, respectively, bias of 34 V (for which we measured a lateral and vertical etch rates of 1 and 3 nm s −1 , respectively). A step of Ar plasma was introduced to remove the oxidized top of the tungsten film from the trenches, thus exposing metallic tungsten. The latter was used as electrode for the electroplating of a 40-nm-thick Ni film in a Watts bath at 56 °C. The array of resist pillars was stripped in acetone, leaving an array of holes in the electroplated Ni film. The pattern was transferred in a single step into the W film and into Si by dry etching in an inductively coupled plasma reactor. For the γ- series, a Bosch process with 12 cycles of passivation/etching was used to form deep trenches with periodic restriction (‘scallops’). The 10-s duration passivation steps were carried out in a flux of C 4 F 8 and Ar at 100 and 20 s.c.c.m., respectively, and 600 W applied RF power to the coil only. The 18-s etching steps were done in a flux of SF 6 and Ar at 100 and 20 s.c.c.m., respectively, and 50/600 W RF power to the platen and coil. Sample γ 1 was taken out from the batch and tungsten was wet etched in boiling H 2 O 2 , resulting in the lift-off of the nickel mask. For the δ -series, the etching parameters were 8 mTorr pressure, C 4 F 8 , SF 6 and Ar gas flows of 60, 30 and 10 s.c.c.m., respectively, and 400 and 20 W coil and platen RF power, respectively. Samples δ 1 and ω (the latter with an additional step of wet etching of tungsten in boiling H 2 O 2 for lifting the mask) were taken out from the batch at this stage for measurement. Samples δ 2 , δ 3 , δ 4 and γ 2 were further processed. The holes obtained after plasma etching with imperfect profile were further etched by wet anisotropic etching in tetramethylammonium hydroxide 25%w aqueous solution, at a temperature of 60 °C for 35 s under stirring condition. The process resulted in the formation of holes delimited by {111} planes. The sample δ 2 was taken out from the batch at this stage for measurement. The tungsten layer in samples δ 3 , δ 4 and γ 2 was etched by wet etching in boiling hydrogen peroxide (H 2 O 2 ), lifting the nickel mask above it. The sample δ 3 was taken out at this stage from the batch for measurement. The bottleneck presents at the top of the holes (formed by the planes and ) was removed from samples δ 4 and γ 2 by spin coating a film of polymethyl methacrylate to protect the holes. Next, the resist was etched back by oxygen plasma until the top of the silicon surface was exposed. Further, the silicon substrate was etched with a plasma of C 4 F 8 , SF 6 and Ar at flows of 60, 30 and 10 s.c.c.m., respectively, and 400 and 20 W RF power to the coil and platen, respectively, for 20 s. Finally, the polymethyl methacrylate was dissolved in warm acetone, leaving holes without bottleneck. Characterization of the samples A statistics of the main geometrical parameters characterizing the pores in the different samples was obtained by SEM, using a Zeiss Supra 40 at 10 kV acceleration voltage. Twenty images were taken in top view at random positions on the surface of each sample with the same magnification of × 70K. For each image, one pore (the central one in the image) was characterized. The mean value and s.d. were calculated for all geometrical parameters. The measure of the parameters obtained from the cross-sectional view was obtained by selecting a few representative images, where the cleavage of the sample was cutting approximately in the middle the pores. The statistics for the parameters obtained from cross-view images was done by averaging five to ten values and it is summarized in Supplementary Table S1 . We have also estimated an upper limit for the roughness of the inner surface of the pores. In principle, this could be achieved by scanning probes techniques (atomic force or scanning tunnelling microscopy) on single pores’ cross-section. However, because of the recession and the high curvature of the cross-sectioned pores’ surface, the useful scanning range of the tip would be only a few tens of nanometres. Therefore, we used a different approach, based on the assumption that the nanoscale protrusions that are present at the surface of the ‘rough’ samples (that is, γ 1 , δ 1 , ω , which were etched only by a dry process) could be approximated by hemispheres. Using Gwyddion, a programme for the analysis of scanning probe images, the statistical distribution of ‘particle’ diameters inside the pores was obtained for a few representative pores, from SEM images taken at high magnification. Using the assumption that the height is equal to the equivalent radius for any identified particle, an upper limit of 3 nm (r.m.s.) for the surface roughness was obtained for the three samples γ 1 , δ 1 and ω . For sample γ 1 , the scallops were considered real geometrical features and not roughness. As such, the ridges were excluded from the computation of the surface roughness. For all other samples whose surface was smoothed by the wet etching step, we could not appreciate the presence of features that could be analysed as particles and we guess that the r.m.s. roughness is well below 1 nm. As for the surface wall chemistry, we have to distinguish between the samples that underwent only plasma etching and those that were etched also in the alkaline solution (KOH in water) after plasma etching. The chemical functionalities of the surfaces are in fact different. In the case of the dry etching, a very thin passivation layer of fluorocarbons remains on the surface. In the case of wet etching, a hydrogen-terminated silicon surface remains at the end of the process. In both cases, the surface is chemically uniform and no variations in the fluid/wall interaction are expected. The different surface energy of the dry- and wet-etched samples does not lead to any appreciable difference in the adsorption isotherms, because liquid argon completely wet both surfaces. Adsorption measurements The adsorption has been measured with a torsional oscillator. The sample is attached to the extremity of a hardened steel rod and is driven to the torsional resonant frequency of the system: where K is the elastic constant and I is the total moment of inertia. A schematic drawing of the torsional disk oscillator used in the measurements is shown in Fig. 1C . As the substrate is exposed to a vapour, the resonance frequency changes because of a variation in the moment of inertia Δ I all . If I 0 and f 0 indicate the moment of inertia and the resonance frequency in vacuum, respectively, then where f is the oscillator frequency measured at a certain vapour pressure P . The relative increase Δ I all / I 0 is caused by the mass of the adsorbed film and by the hydrodynamic contribution due to the mass of the dynamically displaced fluid. For a thin disk, the frequency decrease due to this viscous coupling has the form [32] : where C and c are two factors, which take into account the geometry of the sample and the fluid properties. The value of these constants is deduced from a least-squares fitting of the experimental data of the adsorption isotherm for relative pressures P/P 0 ≤0.2, where the frequency decrease is mainly due to viscous coupling [32] . The mass of the adsorbed film is then proportional to the relative change of the oscillator moment of inertia Δ I / I 0 as deduced from the vapour-corrected oscillator frequency . This implies that the resulting adsorption at very low pressures is practically zero. Accordingly, the seeming weak-binding character of the substrate is only an artefact of the analysis method. How to cite this article: Mistura, G. et al. Continuous adsorption in highly ordered porous matrices made by nanolithography. Nat. Commun. 4:2966 doi: 10.1038/ncomms3966 (2013).